Pirt functions as an endogenous regulator of TRPM8 Pirt is a membrane protein that is specifically expressed in the peripheral nervous system, where it has been shown to increase the sensitivity of the transient receptor potential vanilloid 1 channel and modulate its role in heat pain. The broad expression of Pirt among dorsal root ganglion neurons suggests it may modulate other transient receptor potentials, such as the menthol and cooling sensor TRPM8. The discrepancies in the channel properties of TRPM8 in native neurons versus heterologous cells indicate the existence of endogenous modulators of the channel. Here we show that Pirt regulates the function of TRPM8 and its role in detecting cold. Pirt −/− mice exhibit decreased behavioural responses to cold and cool temperatures, and Pirt increases the sensitivity of TRPM8 to menthol and cool temperature. Our data suggest Pirt is an endogenous regulator of TRPM8. Tsavaler et al. [1] first identified the Trp-p8 gene from a human prostate-specific complementary DNA (cDNA) library and proposed that it may be an ion channel with oncogene or tumour promoter potential. The same gene was later identified as a cold-activated channel by two independent groups [2] , [3] . They discovered that Trp-p8 encodes a Ca 2+ -permeable ion channel that is activated by cold and by cooling agents such as menthol, eucalyptol and icilin. Following the unified nomenclature for transient receptor potential (TRP) channels, Trp-p8 was classified as part of the TRP melastatin (TRPM) subfamily and renamed TRPM8 (refs 4 , 5 ). TRPM8 is known for two roles, cooling and analgesia, as low doses of menthol induce a sensation of cooling and analgesia in inflammatory (complete Freund’s Adjuvant model) and neuropathic (chronic constriction injury model) pain models [6] . Much higher doses of menthol induce a noxious cold sensation [7] , although it is not clear if TRPM8 is specifically being targeted at such doses. Notably, the threshold temperatures of recombinant TRPM8 channels are consistently lower than those of native channels in menthol-sensitive trigeminal neurons, which suggests that temperature sensitivity is facilitated by endogenous factors in vivo [8] , [9] . Besides temperature and cooling agents, a number of factors are known to regulate TRPM8, such as pH [10] and phospholipids [11] , [12] . Single-channel recording has been used to investigate whether the regulation of TRPM8 occurs through the modulation of channel properties. For example, Zakharian et al. [13] showed that phosphatidylinositol 4,5-bisphosphate (PIP 2 ) participates in the gating of TRPM8. However, there is still a dearth of information about the mechanisms that regulate TRPM8, especially in the context of detecting cool temperatures or cooling agents. A recently discovered gene named Pirt encodes a two-transmembrane domain protein that is specifically expressed in peripheral sensory neurons. Pirt binds to both PIP 2 and transient receptor potential vanilloid 1 (TRPV1) and is necessary for the PIP 2 -dependent activation of TRPV1 (ref. 14 ). It regulates the physiological function of TRPV1 and contributes to both histamine-dependent and -independent itch [14] , [15] . As Pirt is widely expressed in primary sensory neurons in dorsal root ganglion (DRG) beyond just TRPV1-positive neurons (that is, most if not all small- to medium-diameter neurons), it is highly possible that Pirt regulates other TRP channels. Our previous data have shown that Pirt does not bind to TRPA1 (ref. 14 ). Furthermore, both loss-of-function and gain-of-function studies suggest that Pirt does not modulate TRPA1 (ref. 14 ). However, Pirt does bind to TRPM8 (ref. 14 ), and this observation together with the difference in the properties of recombinant TRPM8 versus TRPM8 in native DRG neurons raise an interesting possibility that Pirt may function as an endogenous regulator of TRPM8. In this study, we used calcium imaging and electrophysiology to demonstrate that Pirt enhances TRPM8 channel properties, including temperature threshold and menthol sensitivity. Pirt −/− (knockout, KO) mice show impaired behavioural responses to cold and cool temperature and chemical agents compared with wild-type (WT) mice. Therefore, Pirt is an endogenous positive regulator of TRPM8 in addition to modulating TRPV1. Pirt −/− mice exhibit impaired cold sensitivity To assess the possible involvement of Pirt in cold nociception, we performed several cold nociceptive behaviour experiments using Pirt −/− mice and WT littermates. In the cold plate (−1 °C) experiment, the latency for a mouse to withdraw its paw from the cold plate was measured. Pirt −/− mice exhibited significantly longer paw-withdrawal latencies (21.2±1.3 s) compared with WT control mice (15.8±1.3 s, P =0.005, Fig. 1a ). A previous study has shown that icilin evokes cold hyperalgesia in a TRPM8-dependent manner [16] . With the cold plate set to 0 °C, icilin (10 μl, 2.4 mg ml −1 ) was injected into the hindpaw, and the observed paw-withdrawal latency was also significantly prolonged in Pirt −/− mice (16.1±2.1 s, 15 min after icilin injection) compared with WT mice (4.3±0.6 s, P <0.0001, Fig. 1b ). Besides noxious cold, TRPM8 is also essential for mice to sense and avoid cool temperature. Trpm8 −/− mice lose the ability to discriminate cool temperature from room or warm temperature during the thermal preference test [16] , [17] , [18] . To investigate the role of Pirt in recognizing cool temperature, we performed the thermal preference test on Pirt −/− and WT mice (preferring 32 °C chamber over 15 °C chamber). To examine how the animals’ avoidance of the cool temperature trended throughout the 60-min time course, we plotted the percentage of time spent at 15 °C chamber in 5 min intervals ( Fig. 1c , left panel). Interestingly, WT mice gradually avoided the cool temperature as the 60 min passed. Pirt KO mice did not exhibit a similar time-dependent avoidance (at least not in the early phase). Using a two-way analysis of variance test with Bonferroni correction for repeated measure showed that the difference in the time course measurement between the two groups is highly significant ( P <0.0001, n =12 for each genotype). We also compared cumulative time spent at 15 °C over the 60-min time course. Although there is a trend, the difference did not reach statistical significance ( P =0.12; Fig. 1c , right panel). Together, these data suggest that Pirt has a role in noxious cold and cool temperature sensation. 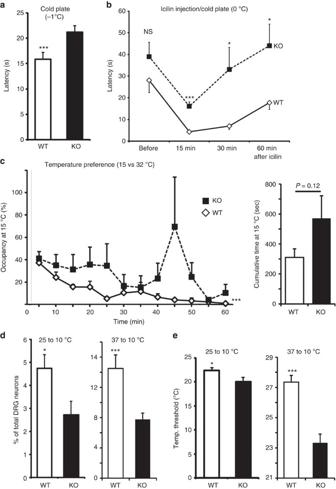Figure 1:Pirt−/−mice demonstrate impaired behavioural and cellular responses to cold and cool temperature. (a) Paw-withdrawal latencies of mice in the cold plate (−1 °C) experiment.Pirt−/−mice (KO) have increased latencies (21.2±1.3 s,n=12) compared with WT littermates (15.8±1.3 s,n=11, ***P=0.005, two-tailed unpaired Student’st-test). (b) Icilin-evoked cold hyperalgesia in the cold plate (0 °C) experiment. Fifteen min after icilin injection (10 μl of 2.4 mg ml−1), the latency is significantly prolonged inPirt−/−(16.1±2.1 s) versus WT (4.3±0.6 s; 17 mice per genotype; *P<0.05, ***P<0.0001, two-tailed unpaired Student’st-test) mice. (c) Two-temperature preference assay (32 °C versus 15 °C). Individual freely moving WT andPirt−/−mouse (12 mice per genotype) was placed in a chamber with floors at either 32 °C or 15 °C. Left panel: percentage of time spent at each temperature-controlled floors was monitored for 5 min intervals over 60 min. ***P<0.0001, two-way analysis of variance with repeated measures. Right panel: cumulative time spent at 15 °C over 60 min.P=0.12, two-tailed unpaired Student’st-test. (d,e) Calcium responses of cultured DRG neurons to cooling (25–10 °C and 37–10 °C, left and right columns, respectively). More than 600 neurons from three animals of each genotype per cooling condition were analysed. (d) FewerPirt−/−than WT DRG neurons responded to cooling. (e) Cold temperature threshold of activation in DRG neurons. The threshold for evoking a calcium response was significantly lower inPirt−/−neurons compared with WT neurons. *P<0.05, ***P<0.0001, two-tailed unpaired Student’st-test for panelsdande. Error bars represent s.e.m. NS, nonsignificant. Figure 1: Pirt −/− mice demonstrate impaired behavioural and cellular responses to cold and cool temperature. ( a ) Paw-withdrawal latencies of mice in the cold plate (−1 °C) experiment. Pirt −/− mice (KO) have increased latencies (21.2±1.3 s, n =12) compared with WT littermates (15.8±1.3 s, n =11, *** P =0.005, two-tailed unpaired Student’s t -test). ( b ) Icilin-evoked cold hyperalgesia in the cold plate (0 °C) experiment. Fifteen min after icilin injection (10 μl of 2.4 mg ml −1 ), the latency is significantly prolonged in Pirt −/− (16.1±2.1 s) versus WT (4.3±0.6 s; 17 mice per genotype; * P <0.05, *** P <0.0001, two-tailed unpaired Student’s t -test) mice. ( c ) Two-temperature preference assay (32 °C versus 15 °C). Individual freely moving WT and Pirt −/− mouse (12 mice per genotype) was placed in a chamber with floors at either 32 °C or 15 °C. Left panel: percentage of time spent at each temperature-controlled floors was monitored for 5 min intervals over 60 min. *** P <0.0001, two-way analysis of variance with repeated measures. Right panel: cumulative time spent at 15 °C over 60 min. P =0.12, two-tailed unpaired Student’s t -test. ( d , e ) Calcium responses of cultured DRG neurons to cooling (25–10 °C and 37–10 °C, left and right columns, respectively). More than 600 neurons from three animals of each genotype per cooling condition were analysed. ( d ) Fewer Pirt −/− than WT DRG neurons responded to cooling. ( e ) Cold temperature threshold of activation in DRG neurons. The threshold for evoking a calcium response was significantly lower in Pirt −/− neurons compared with WT neurons. * P <0.05, *** P <0.0001, two-tailed unpaired Student’s t -test for panels d and e . Error bars represent s.e.m. NS, nonsignificant. Full size image After observing the deficit in the behavioural responses to cold in Pirt −/− mice, we tested whether a corresponding cellular deficit was present. In cultured DRG neurons, we used calcium imaging to compare the proportion of WT and Pirt −/− cells that responded to cold. Cooling the bath temperature from 25 to 10 °C evoked a calcium response in 4.8% of DRG neurons cultured from WT mice versus 2.7% of neurons from Pirt −/− mice ( P <0.05, Fig. 1d , left columns). Furthermore, the temperature threshold for evoking a calcium response was significantly lower in Pirt −/− (20.0±0.9 °C) than in WT neurons (22.4±0.5 °C, P <0.05, Fig. 1e , left columns). To study the role of Pirt in a more physiological temperature range and avoid desensitization of TRPM8, we employed another cooling paradigm to evoke DRG neuron activation monitored by calcium imaging. Indeed, the deficit of Pirt −/− DRG neurons in response to cooling is more dramatic when warmer temperatures were used and the bath temperature was decreased from 37 to 10 °C compared with the response induced by cooling from 25 to 10 °C. Cooling from 37 to 10 °C evoked a calcium response in 14.5% of WT DRG neurons, whereas 7.7% of Pirt −/− neurons responded ( P <0.005, Fig. 1d , right columns). The temperature threshold to activate Pirt −/− neurons was significantly lower (23.3±0.6 °C) than that of WT neurons (27.4±0.4 °C, P <0.005, Fig. 1e , right columns). The cellular phenotypes, which suggest an impaired sensitivity of Pirt −/− DRG neurons to cold temperature, are in agreement with the behavioural data showing that Pirt −/− mice have diminished responses to noxious cold and impaired ability to sense cool temperature. Pirt specifically enhances TRPM8-mediated calcium influx We performed calcium imaging experiments in Fura 2-AM-loaded human embryonic kidney (HEK) 293 cells that transiently expressed TRPM8 and Pirt, or TRPM8 alone ( Fig. 2a ). In a randomly chosen visual field, a variable proportion of cells (5–80%) responded to cooling (from 37 to 18 °C) or to the application of menthol (3–3,000 μM). During cooling, TRPM8-expressing cells began to respond with an increase in the intracellular Ca 2+ concentration at 21.2 °C and were half-maximally activated (T 50 ) at 14.6 °C ( n =63). The activation properties of cells coexpressing TRPM8 and Pirt were significantly shifted to warmer temperatures: the threshold was 23.8 °C ( P <0.001) and the T 50 was 16.7 °C ( n =66, P <0.001, Fig. 2b ). In addition, the mean amplitude of the cooling-induced Ca 2+ signals was higher in the TRPM8- and Pirt-coexpressing cells (0.58±0.04, n =66) than in the cells expressing TRPM8 alone (0.36±0.07, n =63, P <0.01; Fig. 2c ). These data are in agreement with our hypothesis that Pirt sensitizes TRPM8 to cold detection and augments TRPM8-mediated cold signalling. 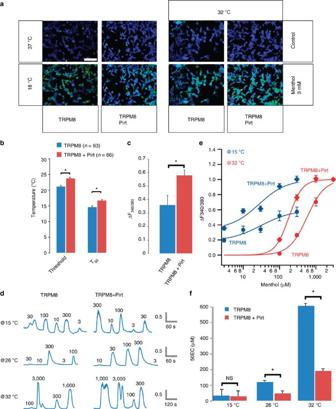Figure 2: Pirt enhances TRPM8-mediated calcium influx. (a) Calcium imaging of Fura-2-AM-loaded HEK293 cells. Cells expressing TRPM8 and Pirt showed calcium responses to cooling (18 °C) and menthol (3 mM, 32 °C). The scale bar represents 100 μm. (b) Temperature threshold of activation and half-maximal temperature of activation (T50) of TRPM8 alone or coexpressed with Pirt. The presence of Pirt increases the temperature threshold to 23.8 °C (n=66) compared with TRPM8 alone (21.2 °C,n=63, *P<0.001, two-tailed unpaired Student’st-test). Pirt also shifts the T50to 16.7 °C from 14.6 °C with TRPM8 alone (*P<0.001, two-tailed unpaired Student’st-test). (c) Amplitude of cooling-induced Ca2+signals. The mean amplitude of the calcium response (ΔF340/F380 ratio) is higher in the presence of Pirt (0.58±0.04;n=66) than in its absence (0.36±0.07,n=63, *P<0.01, two-tailed unpaired Student’st-test). (d) Representative calcium signals from the application of menthol (3, 10, 30, 100, 300, 1,000 and 3,000 μM) to TRPM8- or TRPM8- and Pirt-expressing cells at cool (15 °C), ambient (26 °C) and warm (32 °C) temperatures. The order in which the various menthol concentrations were applied was permuted to prevent bias from desensitization. (e) Concentration–response curves for menthol at 32 and 15 °C. (f) The apparent affinity (EC50) of TRPM8 for menthol differs in presence or absence of recombinant Pirt and is dependent on the temperature. The EC50for menthol at 32 °C was found to be 180±16 μM in the presence (n=100) and 570±17 μM in the absence of Pirt (n=126; *P=0.017, two-tailed unpaired Student’st-test). At 26 °C, the menthol EC50is 45±18 μM in the presence and 113±5 μM in the absence of Pirt (*P=0.005, two-tailed unpaired Student’st-test). TRPM8 is already activated by cooling at 15 °C, but still shows a dependence on menthol concentration (EC50values: TRPM8/Pirt, 27±29 μM, TRPM8, 31±39 μM (P=0.094). Error bars represent s.e.m. NS, nonsignificant. Figure 2: Pirt enhances TRPM8-mediated calcium influx. ( a ) Calcium imaging of Fura-2-AM-loaded HEK293 cells. Cells expressing TRPM8 and Pirt showed calcium responses to cooling (18 °C) and menthol (3 mM, 32 °C). The scale bar represents 100 μm. ( b ) Temperature threshold of activation and half-maximal temperature of activation (T 50 ) of TRPM8 alone or coexpressed with Pirt. The presence of Pirt increases the temperature threshold to 23.8 °C ( n =66) compared with TRPM8 alone (21.2 °C, n =63, * P <0.001, two-tailed unpaired Student’s t -test). Pirt also shifts the T 50 to 16.7 °C from 14.6 °C with TRPM8 alone (* P <0.001, two-tailed unpaired Student’s t -test). ( c ) Amplitude of cooling-induced Ca 2+ signals. The mean amplitude of the calcium response (ΔF340/F380 ratio) is higher in the presence of Pirt (0.58±0.04; n =66) than in its absence (0.36±0.07, n =63, * P <0.01, two-tailed unpaired Student’s t -test). ( d ) Representative calcium signals from the application of menthol (3, 10, 30, 100, 300, 1,000 and 3,000 μM) to TRPM8- or TRPM8- and Pirt-expressing cells at cool (15 °C), ambient (26 °C) and warm (32 °C) temperatures. The order in which the various menthol concentrations were applied was permuted to prevent bias from desensitization. ( e ) Concentration–response curves for menthol at 32 and 15 °C. ( f ) The apparent affinity (EC 50 ) of TRPM8 for menthol differs in presence or absence of recombinant Pirt and is dependent on the temperature. The EC 50 for menthol at 32 °C was found to be 180±16 μM in the presence ( n =100) and 570±17 μM in the absence of Pirt ( n =126; * P =0.017, two-tailed unpaired Student’s t -test). At 26 °C, the menthol EC 50 is 45±18 μM in the presence and 113±5 μM in the absence of Pirt (* P =0.005, two-tailed unpaired Student’s t -test). TRPM8 is already activated by cooling at 15 °C, but still shows a dependence on menthol concentration (EC 50 values: TRPM8/Pirt, 27±29 μM, TRPM8, 31±39 μM ( P =0.094). Error bars represent s.e.m. NS, nonsignificant. Full size image After analysing the effect of Pirt expression on the temperature sensitivity of TRPM8, we were interested in a possible modulatory effect of Pirt on the sensitivity of TRPM8 to menthol. To investigate this possibility, we applied various concentrations of menthol (3–3,000 μM) to TRPM8- or TRPM8- and Pirt-expressing HEK293 cells at warm (32 °C), ambient (26 °C) or cold (15 °C) temperatures ( Fig. 2d–f ). To prevent any bias of the concentration–response relationship from the desensitization of TRPM8-mediated Ca 2+ signals following repetitive menthol application, we did not exclusively apply menthol in ascending or descending concentrations; rather, we permuted the sequence of consecutive applications. Analysing the peak amplitudes of the Ca 2+ signals induced by different concentrations of menthol in the six groups, we found an apparent affinity (EC 50 ) of 570±17 μM for TRPM8 at 32 °C, which was significantly reduced to 180±16 μM when Pirt was coexpressed ( Fig. 2f ). When cooling to 15 °C, the TRPM8 receptors were already activated by temperature, but they still showed a clear dependence on the menthol concentration ( Fig. 2e ). The EC 50 values were estimated to be 27±29 μM for TRPM8/Pirt and 31±39 μM for TRPM8-expressing cells. However, at a given menthol concentration, the mean Ca 2+ signals in TRPM8- and Pirt-coexpressing HEK293 cells were significantly larger than in cells expressing only TRPM8. These data indicate that the apparent affinity of TRPM8 for menthol is clearly increased by the presence of Pirt under ambient and warm conditions but not during cooling, when TRPM8 is already sensitized to menthol by the action of cold temperature. Pirt enhances TRPM8-mediated currents We performed whole-cell voltage-clamp recordings to investigate whether Pirt can increase TRPM8-mediated currents at room temperature (~25 °C). We applied various concentrations of menthol (0.1–1,000 μM) to challenge cells expressing TRPM8 and Pirt or TRPM8 alone. We found the modulatory effect of Pirt on TRPM8 to be concentration-dependent. At menthol concentrations below 5 μM, the menthol-induced currents were hardly detectable and did not differ between cells expressing TRPM8 and Pirt or TRPM8 alone ( Fig. 3a ). Menthol concentrations greater than 5 μM evoked currents that had increased amplitudes with increasing menthol concentrations, reaching a maximum amplitude at 1 mM menthol. The current density, calculated from the amplitudes of the menthol responses corrected for the capacitance of the recorded cells, was significantly higher in cells expressing TRPM8 and Pirt compared with cells expressing TRPM8 alone ( Fig. 3a ). The menthol concentration–response curve was shifted to lower concentrations in the presence of Pirt ( Fig. 3a ) and revealed EC 50 values of 87.3±1.3 μM menthol for TRPM8/Pirt and 150.9±3.57 μM for TRPM8 alone. The latter value is similar to the data from a previous report that determined the EC 50 in heterologous cells to be 124 μM (ref. 19 ). 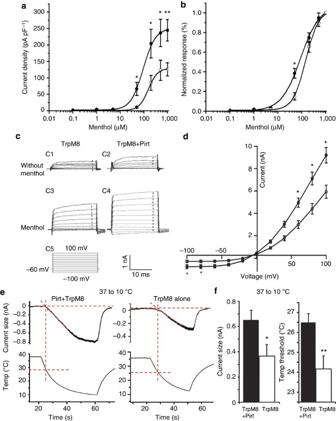Figure 3: Pirt enhances TRPM8 currents evoked by menthol and cold temperature. (a) Menthol dose–response curves of TRPM8-expressing cells transfected with (closed circles) or without Pirt (open circles). When 50, 200, 500 or 1,000 μM menthol was applied to TRPM8/Pirt and TRPM8 alone, respectively, the current density was significantly different (*P<0.05,n=7 and 7 at 50 μM,n=13 and 13 at 200 μM,n=17 and 17 at 500 μM; **P<0.01,n=37 and 34 at 1,000 μM; two-tailed unpaired Student’st-test). The EC50values for TRPM8+Pirt and TRPM8 alone were 87.31±1.3 and 150.94±3.57 μM, respectively. (b) Normalized concentration–response relationship. The TRPM8/Pirt curve was shifted to the left of TRPM8 alone, and the EC50values were 89.85±7.36 and 147.75±7.19 μM, respectively. (c) Representative current traces of TRPM8 and TRPM8/Pirt with and without menthol. The left (C1 and C3) and right (C2 and C4) traces indicate TRPM8 alone and TRPM8/Pirt, respectively. The upper (C1 and C2) and lower (C3 and C4) traces indicate the absence and presence of menthol, respectively. The C5 trace indicates the voltage step protocol. (d) Voltage–current relationship curves of TRPM8 with (closed circles) and without (open circles) Pirt constructed from currents in the presence of menthol (1 mM) with background currents subtracted (TRPM8/Pirt,n=27, TRPM8 alone,n=28; *P<0.05; two-tailed unpaired Student’st-test). (e) Cold-evoked current traces in the TRPM8/Pirt (top left) and TRPM8 alone (top right) groups. The bottom traces show the application of cold buffer 37–10 °C. Temperature thresholds were determined by the corresponding temperature point where the slope of current rise intercepted with the current baseline. (f) Left columns: cold temperature-evoked average current size of TRPM8 with (black bar) and without (white bar,n=16 per group) Pirt. Right columns: cold-evoked temperature threshold of TRPM8/Pirt (black bar) or TRPM8 alone (white bar,n=16 per group). *P<0.05, **P<0.01, two-tailed unpaired Student’st-test. Error bars represent s.e.m. Figure 3: Pirt enhances TRPM8 currents evoked by menthol and cold temperature. ( a ) Menthol dose–response curves of TRPM8-expressing cells transfected with (closed circles) or without Pirt (open circles). When 50, 200, 500 or 1,000 μM menthol was applied to TRPM8/Pirt and TRPM8 alone, respectively, the current density was significantly different (* P <0.05, n =7 and 7 at 50 μM, n =13 and 13 at 200 μM, n =17 and 17 at 500 μM; ** P <0.01, n =37 and 34 at 1,000 μM; two-tailed unpaired Student’s t -test). The EC 50 values for TRPM8+Pirt and TRPM8 alone were 87.31±1.3 and 150.94±3.57 μM, respectively. ( b ) Normalized concentration–response relationship. The TRPM8/Pirt curve was shifted to the left of TRPM8 alone, and the EC 50 values were 89.85±7.36 and 147.75±7.19 μM, respectively. ( c ) Representative current traces of TRPM8 and TRPM8/Pirt with and without menthol. The left (C1 and C3) and right (C2 and C4) traces indicate TRPM8 alone and TRPM8/Pirt, respectively. The upper (C1 and C2) and lower (C3 and C4) traces indicate the absence and presence of menthol, respectively. The C5 trace indicates the voltage step protocol. ( d ) Voltage–current relationship curves of TRPM8 with (closed circles) and without (open circles) Pirt constructed from currents in the presence of menthol (1 mM) with background currents subtracted (TRPM8/Pirt, n =27, TRPM8 alone, n =28; * P <0.05; two-tailed unpaired Student’s t -test). ( e ) Cold-evoked current traces in the TRPM8/Pirt (top left) and TRPM8 alone (top right) groups. The bottom traces show the application of cold buffer 37–10 °C. Temperature thresholds were determined by the corresponding temperature point where the slope of current rise intercepted with the current baseline. ( f ) Left columns: cold temperature-evoked average current size of TRPM8 with (black bar) and without (white bar, n =16 per group) Pirt. Right columns: cold-evoked temperature threshold of TRPM8/Pirt (black bar) or TRPM8 alone (white bar, n =16 per group). * P <0.05, ** P <0.01, two-tailed unpaired Student’s t -test. Error bars represent s.e.m. Full size image To investigate a possible effect of Pirt on the voltage dependence of TRPM8, we measured current–voltage relationships for menthol-evoked currents in HEK293 cells expressing TRPM8 and Pirt or TRPM8 alone. In the presence of 1 mM menthol, we applied voltage steps ranging from −100 to +100 mV ( Fig. 3c ). At negative voltages, only small inward currents were recorded, and the current amplitudes were significantly larger in the presence of Pirt at −100 and −80 mV compared with cells expressing TRPM8 alone. However, at positive voltages, large outward currents were evoked, showing significant differences between TRPM8- and Pirt-expressing versus TRPM8-expressing cells at positive potentials ranging from +60 to +100 mV. We then co-transfected TRPM8 with a non-functional mutant form of Pirt, in which the positively charged amino acids in the C terminus were changed to neutral residues [14] . No differences in the current amplitudes between the TRPM8/Pirt mutant and TRPM8 groups were detected ( Fig. 4 ). We also tested the role of the Pirt C terminus by coexpressing TRPM8 with a glutathione S -transferase-tagged form of the Pirt C terminus in HEK293 cells. It significantly enhanced menthol-evoked currents compared with control cells coexpressing TRPM8 and glutathione S -transferase ( Fig. 4 ). Together, these results indicate that the presence of Pirt is sufficient to enhance TRPM8-mediated currents and that the positively charged amino acids residing in the C terminus of Pirt are key components involved in mediating this effect. 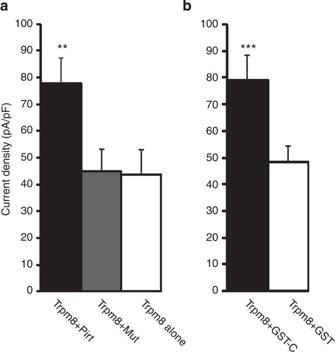Figure 4: The intact Pirt C terminus is required for TRPM8 modulation. (a) Menthol (1 mM)-evoked currents in HEK293 cells transfected with TRPM8. The coexpression of Pirt increases the current intensity of TRPM8 (black bar,n=19) compared with the control group (white bar,n=15; **P<0.001 two-tailed unpaired Student’st-test), but the Pirt mutant, with the positively charged amino acids in its C terminus replaced with neutral residues, has no effect (grey bar,n=14). (b) Menthol-evoked currents of TRPM8 with glutathioneS-transferase (GST; white bar,n=23) and Pirt GST-C (black bar,n=24). The C terminus of Pirt significantly enhances TRPM8 current. ***P<0.005 two-tailed unpaired Student’st-test. Error bars represent s.e.m. Figure 4: The intact Pirt C terminus is required for TRPM8 modulation. ( a ) Menthol (1 mM)-evoked currents in HEK293 cells transfected with TRPM8. The coexpression of Pirt increases the current intensity of TRPM8 (black bar, n =19) compared with the control group (white bar, n =15; ** P <0.001 two-tailed unpaired Student’s t -test), but the Pirt mutant, with the positively charged amino acids in its C terminus replaced with neutral residues, has no effect (grey bar, n =14). ( b ) Menthol-evoked currents of TRPM8 with glutathione S -transferase (GST; white bar, n =23) and Pirt GST-C (black bar, n =24). The C terminus of Pirt significantly enhances TRPM8 current. *** P <0.005 two-tailed unpaired Student’s t -test. Error bars represent s.e.m. Full size image Because the behavioural experiments with Pirt −/− mice indicate that the absence of Pirt dampens responsiveness in the cold plate test, we examined whether Pirt changes the temperature threshold of cooling stimulation. We transfected Pirt and TRPM8 cDNA into HEK293 cells and measured the temperature-induced currents and temperature threshold in response to cold temperature in TRPM8- and Pirt- versus TRPM8-expressing cells. We observed inward currents when the temperature was reduced from 37 °C to approximately 10 °C ( Fig. 3e ). The size of cold temperature-evoked current in TRPM8/Pirt cells was significantly larger than that of cells with TRPM8 alone (650.6±77.2 versus 364.8±92.2 pA, P <0.05, n =16; Fig. 3f ). The TRPM8/Pirt cells also exhibited a significantly higher temperature threshold than the TRPM8 cells (26.5±0.4 °C versus 24.2±0.4 °C, P <0.01, n =16; Fig. 3f ). To rule out a possible effect of Pirt on TRPM8 protein expression, we performed western blot analysis and found that the coexpression of Pirt did not alter the total protein levels or cell-surface expression of TRPM8 in HEK293 cells ( Fig. 5 and Supplementary Fig. S1 ). 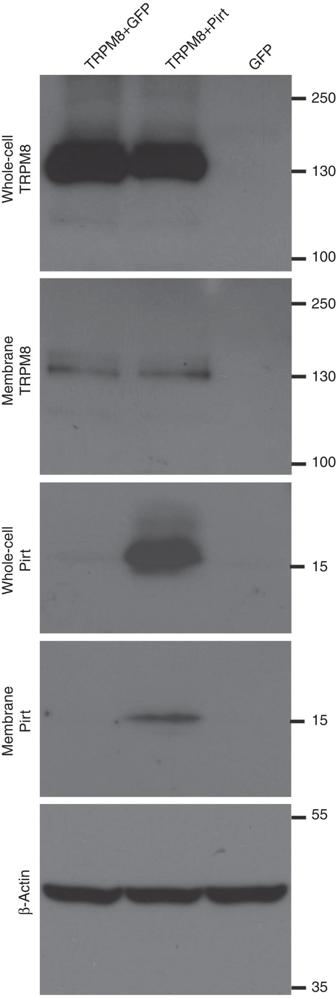Figure 5: Coexpression of Pirt does not influence the expression of TRPM8. The expression level of TRPM8–myc in HEK293 cells was measured by western blot after plasma membrane proteins were biotinylated and purified with streptavidin. β-Actin was used as a loading control. The expression of TRPM8 (probed with an anti-myc antibody) in whole-cell lysates (whole-cell TRPM8) or cell surface (membrane TRPM8) are at similar levels whether or not Pirt (probed with an anti-Pirt antibody) is coexpressed. The specificity of TRPM8 band was determined by the absence of the band in samples from HEK293 cells transfected with GFP alone. The molecular markers (kD) are indicated at the right side of the blots. Figure 5: Coexpression of Pirt does not influence the expression of TRPM8. The expression level of TRPM8–myc in HEK293 cells was measured by western blot after plasma membrane proteins were biotinylated and purified with streptavidin. β-Actin was used as a loading control. The expression of TRPM8 (probed with an anti-myc antibody) in whole-cell lysates (whole-cell TRPM8) or cell surface (membrane TRPM8) are at similar levels whether or not Pirt (probed with an anti-Pirt antibody) is coexpressed. The specificity of TRPM8 band was determined by the absence of the band in samples from HEK293 cells transfected with GFP alone. The molecular markers (kD) are indicated at the right side of the blots. Full size image Pirt is mainly expressed in the DRG and trigeminal ganglia in the peripheral nervous system and is absent from the central nervous system. In the DRG, the neurons that express Pirt, which include TRPV1-positive cells, span over 85% of total neurons. Most if not all Pirt-negative neurons are large-diameter, NF200 + neurons [14] . Thus, the function of Pirt is not limited to TRPV1-positive neurons, and it may also modulate the function of other ion channels, including other members of the TRP family. Recently, we have shown that Pirt does not modulate TRPA1 function [14] . Here we demonstrate that Pirt positively modulates another TRP, TRPM8. In menthol dose–response curves, the regulation of TRPM8 by Pirt is more apparent at higher doses than at lower ones, especially once the menthol concentration reaches the EC 50 value. The enhanced maximum response of TRPM8 to menthol ( Fig. 3a ) is likely due to the increase in the channel conductance by Pirt, as Pirt does not affect TRPM8 membrane trafficking ( Fig. 5 ). The results of our electrophysiological and calcium imaging experiments also show that Pirt shifts the dose–response curve leftward, indicating that the presence of Pirt renders the TRPM8 channel more sensitive to menthol and to cold temperature. Compared with WT mice, Pirt −/− animals show increased latencies in the cold plate test both at baseline and when pretreated with icilin as well as decreased avoidance to cool temperature. These results demonstrate that the absence of Pirt impairs the behavioural response to noxious cold and cool temperatures. Calcium imaging experiments with HEK293 cells expressing TRPM8 and Pirt or TRPM8 alone revealed a clear interdependence of the modulatory effect of Pirt on both the temperature and menthol concentration. At warm temperatures (32 °C), the sensitivity of TRPM8 to menthol was significantly enhanced in the presence of Pirt, although the maximum amplitude of the calcium signal at saturating menthol concentrations was not clearly affected. The most prominent effect of Pirt was detected at intermediate menthol concentrations under this condition. However, at cold temperatures (15 °C), when TRPM8 is already activated, increasing the menthol concentration still lead to increased calcium signals, which were significantly enhanced in the presence of Pirt across the entire range of menthol concentrations tested. The data favour a modulatory mechanism of Pirt that differentially targets the menthol and cold stimulation of TRPM8. We are aware that a direct comparison of the amplitudes and kinetics of menthol- or cold-induced signals recorded as currents in whole-cell voltage-clamp recordings with calcium signals (ΔF340/F380) in imaging experiments is not feasible. The methodological differences between calcium imaging and voltage-clamp recordings include the different nature of the signals (nonspecific cation current versus change in [Ca 2+ ] i , respectively) and different driving forces (controlled by the amplifier-set holding potential versus free-range and changing according to the activity of the cell, respectively). However, both experimental approaches point to a robust, positive modulatory effect of Pirt on TRPM8-mediated activity. The primary afferent fibres for cold sensitivity can be activated by cool temperatures or noxious cold temperatures [20] , [21] . The specific temperature at which humans discriminate between cool and cold sensation is approximately 15 °C (refs 22 , 23 ), and temperatures below 15 °C are generally perceived as painful [24] . The cooling temperature range in which sensory ganglion cells show strong activation is from 10–20 °C. These neurons also respond to menthol and icilin suggesting that the responses were mediated by TRPM8 (ref. 18 ). It is not clear if menthol specifically targets TRPM8 at all doses. Two previous reports have demonstrated that menthol activates TRPA1 at low doses and inhibits the channel at higher doses [25] , [26] . Low doses of menthol produce a sensation of cooling and analgesia in chronic pain models [6] , and much higher doses produce a noxious burning sensation [7] . Our current and previous results have shown that Pirt modulates the function of TRPM8 but not TRPA1. It is well-documented that a small temperature drop in the noxious cold range (for example, between 0 and −5 °C shown in Fig. 4d of Bautista et al. [17] ) will cause a large decrease in paw response latency. In our case ( Fig. 1 ), lowering one degree from 0 °C to −1 °C, the latency for WT mice decreased from 29 to 16 s. Although Dhaka et al. [16] tested TRPM8 KO mice on a cold plate at −1 °C and found no difference compared with WT mice, Colburn et al. [18] showed that TRPM8 KO mice exhibited a significantly longer latency than WT mice on a 0 °C cold plate. Notably, the paw response latency obtained by Colburn et al. [18] was much shorter than that by Dhaka et al. [16] , even though their cold plates were set at 0 and −1 °C, respectively. Therefore, some of the discrepancies are likely due to differences in the experimental settings of each laboratory such as differences in the materials of cold plates and the accuracy of temperature probes. It is possible that other molecules besides TRPM8 are also sensitive to and mediate noxious cold. Pirt −/− mice showed significantly reduced sensitivity to −1 °C compared with WT controls. The difference in the paw response latency is around 5 s (~16 and 21 s for WT and KO, respectively) for the −1 °C cold plate. For the 0 °C cold plate, the difference in average latency is even larger at 10 s (~29 and 39 s for WT and KO, respectively). However, due to a larger variation in the data, the difference did not reach statistical significance. The insignificant difference in the 0 °C test may be due to the steepness of change in latency versus a small temperature change in the noxious cold range and to other molecules that may be involved in transducing noxious cold signals. PIP 2 acts as a positive modulator of TRPM8’s sensitivity to cold or menthol and prevents channel rundown [27] , [28] . In fact, PIP 2 can also gate the channel in the absence of thermal or chemical stimuli [29] . The positively charged residues in the TRP domain, which is located in the C terminus, participate in the interaction of TRPM8 with membrane-bound PIP 2 . Pirt contains positively charged residues in its C terminus that are important for binding PIP 2 . Our previous work [14] demonstrated that Pirt positively regulates TRPV1 via PIP 2 and Pirt binds to TRPM8 in vitro , suggesting that the regulation of TRPM8 by Pirt may be PIP 2 -mediated and through a physical interaction between the two proteins. Our data indicate that Pirt has a key role in thermal sensation by modulating two essential thermal TRPs, TRPV1 and TRPM8. Disrupting the interaction between Pirt and TRPs may provide a novel way to treat pain. Behavioural assays The behavioural tests were performed by individuals blind to genotype. The mice were 2- to 3-month-old males (20–30 g) that had been backcrossed to C57BL/6 mice for at least five generations. All experiments were performed using a protocol approved by the Animal Care and Use Committee of Johns Hopkins University School of Medicine. Cold plate test was performed as following. A ceramic plate on a bed of ice was cooled in a −20 °C freezer. During the test, the plate was allowed to warm to −1 °C as measured by two independent temperature probes. An individual mouse was placed on the cold plate. The onset of brisk hindpaw lifts and/or flicking/licking of the hindpaw was assessed. For icilin injection/cold plate test, the baseline response was determined before icilin injection, as described above, on a 0 °C cold plate. An aliquot of 10 μl of 2.4 mg ml −1 icilin was injected into one hindpaw of the mouse. Fifteen, 30 and 60 min after icilin injection, the mice were tested for an injected hindpaw response on 0 °C cold plate as described above. Thermal preference assay was performed as following. An individual mouse was placed in a rectangular chamber with four thermally isolated floors. The temperature of two floors was set at 32 °C and the other two were set at 15 °C. Occupancy on each floor was monitored for 1 h by infrared sensors. Cell culture Human embryonic kidney (HEK) 293 cells were obtained from Dr Paul Worley’s laboratory at Johns Hopkins University School of Medicine. The growth medium of HEK293 cells consisted of 90% DMEM, 10% fetal bovine serum, 50 U ml −1 penicillin and 50 μg ml −1 streptomycin-glutamine (Invitrogen). The cells were cultured at 37 °C in the presence of 95% O 2 and 5% CO 2 . The HEK293 cells were co-transfected with mouse TRPM8 (from Dr M. Caterina of Johns Hopkins University School of Medicine), Pirt and enhanced green fluorescent protein (GFP) cDNAs using Lipofectamine 2000 (Invitrogen) according to the manufacturer’s protocol. TRPM8 and GFP cDNA were co-transfected separately as a control. After 18–24 h, the cells were plated on glass coverslips coated with poly-D-lysine, with laminin occasionally used to coat the coverslips after poly-D-lysine treatment. The voltage-clamp recording and calcium imaging experiments were performed after an additional 1–2 days. Dissociated mouse DRG neurons were prepared using the following procedure: a 3- to 4-week-old male or female mouse was anaesthetized with CO 2 asphyxiation. The DRG from all spinal levels were collected in cold DH10 (90% DMEM/F-12, 10% fetal bovine serum, 1% penicillin-streptomycin-glutamine, Gibco) and treated with enzyme solution (5 mg ml −1 dispase and 1 mg ml −1 collagenase type I in Hank’s Balanced Salt Solution without Ca 2+ or Mg 2+ , Gibco) at 37 °C. Following trituration and centrifugation, the cells were resuspended in DH10, and nerve growth factor was added (50 ng ml −1 , Upstate Biotechnology Inc.). The cells were plated on poly-L-lysine- (0.5 mg ml −1 , Biomedical Technologies Inc., Stoughton, MA) and laminin-coated (10 μg ml −1 , Invitrogen) glass coverslips, cultured in an incubator (95% O 2 and 5% CO 2 ) at 37 °C, and used for calcium imaging within 48 h. Western blotting HEK293 cells were transfected with a TRPM8–myc fusion construct in the presence or absence of a Pirt expression construct. After 24 h, the HEK cells were incubated with 1.0 mg ml −1 sulpho-NHS-SS-Biotin (Pierce) in PBS for 30 min at 4 °C. After quenching, cells were lysed in 500 μl of RIPA buffer. Supernatant from cell lysate was added to BSA-blocked ultralink-neutravidin beads (Pierce) and incubated for 2 h. The proteins were eluted from the beads using 2 × SDS–PAGE sample buffer, and western blotting was performed using the anti-myc, anti-Pirt or anti-β-actin antibodies. Calcium imaging The experiments were performed using a ZEISS live-cell imaging setup based on an inverse microscope (Axio Observer Z.1) equipped with Fluar 40 × /1.3 and EC Plan-Neofluar 20 × /0.50 Ph2 objective lenses (ZEISS, Germany). Fura 2-AM-loaded cells (2 μM, 30 min at 37 °C) were illuminated with light of 340 or 380 nm (BP 340/30 HE, BP 387/15 HE) using a fast wavelength switching and excitation device (Lambda DG-4, Sutter Instrument), and fluorescence was detected at 510 nm (BP 510/90 HE and FT 409) using an AxioCam MRm LCD camera (ZEISS). AxioVision 4.8 software (ZEISS) was used to control the hardware and acquire data. The temperature of the solution in the chamber was controlled by means of an in-line solution heater and CL-100 Bipolar Temperature Controller (Warner Instruments) and measured using a thermistor (TempModul S1, ZEISS) placed directly in the chamber near the cells in the visual field. Cold stimulation protocol The bath temperature of the imaging or recording chamber was kept at ~37 °C by an in-line temperature controller (Warner Inc., TC-324B). To provide a cold stimulus, a cooling system (Warner Inc., CL-100) was also connected to the chamber. Rapid cooling was achieved by switching warm to cold perfusion solution via a complete perfusion valve control system (Warner Inc., VC-66CST). The bath temperature was continuously monitored by thermo-probes in the chamber, and the temperature information was sent to analog-to-digital Digidata 1322 (Axon Instruments). The temperature trace was read out by pClamp9.2 software interface and displayed simultaneously on the same windows with the current trace or Ca 2+ transients. The rate of temperature change was approximately 1 °C/ s −1 . After the temperature reached 10 °C, cold perfusion solution was switched back to warm solution. The threshold of temperature was fixed on the cross point of baseline and the tangent of inward current trace. Electrophysiology Whole-cell voltage-clamp recordings were performed in HEK293 cells transfected with TRPM8, Pirt, and GFP or TRPM8 and GFP. The transfected cells were identified using GFP fluorescence, and cells possessing similar fluorescence intensities were selected for recording. Only one HEK293 cell was tested per coverslip. The current measurements were performed with an Axon 700B amplifier and the pCLAMP9.2 software package (Axon Instruments). The electrodes were pulled (Model PP-830, Narishige) from borosilicate glass (WPI Inc.) and had resistances of 2–4 MΩ after filling. The series resistance was usually less than 10 MΩ and was not compensated. All experiments were performed at room temperature (~25 °C) unless otherwise stated. The holding potential was −60 mV, and the current–voltage relationships were obtained in the voltage range from −100 to +100 mV using 20 mV voltage steps that were 20 ms in duration. The HEK293 cells were perfused with extracellular solution consisting of (in mM): NaCl 140, KCl 4, CaCl 2 2, MgCl 2 2, HEPES 10, glucose 5, with pH adjusted to 7.38 using NaOH. The intracellular pipette solution contained (in mM): KCl 135, MgATP 3, Na 2 ATP 0.5, CaCl 2 1.1, EGTA 2, glucose 5, with pH adjusted to 7.38 using KOH and osmolarity adjusted to 300 mOsm using sucrose. Menthol was used as a TRPM8 agonist. It was dissolved in ethanol (100 mg ml −1 ), stored at −20 °C, and diluted with extracellular solution to different concentrations. All of the solutions were applied to the cell at a rate of 0.5 ml min −1 via a gravity-fed perfusion system (VC-6 Six Channel Valve Controller, Warner Instruments). The electrophysiological recordings were performed by one individual blind to genotype. The data are presented as the mean±s.e.m. Statistical comparisons were made using an unpaired Student’s t- test, and the differences were considered significant at P <0.05. How to cite this article: Tang, Z. et al. Pirt functions as an endogenous regulator of TRPM8. Nat. Commun. 4:2179 doi: 10.1038/ncomms3179 (2013).